Cardioprotection by Klotho through downregulation of TRPC6 channels in the mouse heart Klotho is a membrane protein predominantly produced in the kidney that exerts some antiageing effects. Ageing is associated with an increased risk of heart failure; whether Klotho is cardioprotective is unknown. Here we show that Klotho-deficient mice have no baseline cardiac abnormalities but develop exaggerated pathological cardiac hypertrophy and remodelling in response to stress. Cardioprotection by Klotho in normal mice is mediated by downregulation of TRPC6 channels in the heart. We demonstrate that deletion of Trpc6 prevents stress-induced exaggerated cardiac remodelling in Klotho-deficient mice. Furthermore, mice with heart-specific overexpression of TRPC6 develop spontaneous cardiac hypertrophy and remodelling. Klotho overexpression ameliorates cardiac pathologies in these mice and improves their long-term survival. Soluble Klotho present in the systemic circulation inhibits TRPC6 currents in cardiomyocytes by blocking phosphoinositide-3-kinase-dependent exocytosis of TRPC6 channels. These results provide a new perspective on the pathogenesis of cardiomyopathies and open new avenues for treatment of the disease. Klotho is an antiageing protein predominantly produced in the kidney and several other tissues including parathyroid glands and epithelial cells of the choroids plexus [1] . Mice homozygous for a hypomorphic Klotho allele ( kl / kl ) manifest multiple ageing-related phenotypes including skin and muscle atrophy, hyperphosphatemia, osteoporosis and vascular calcification, and die prematurely at around 2–3 months of age. The full-length Klotho protein is a type-1 membrane protein with a large extracellular domain of 952 amino acids in human, a membrane-spanning segment, and a short 11 amino acids intracellular carboxyl terminus [1] . Membranous Klotho associates with fibroblast growth factor (FGF) receptors to form co-receptors for the ligand FGF23, a bone-derived circulating hormone that lowers serum phosphate levels by increasing renal phosphate excretion, suppressing 1,25-dihyroxyvitamin D synthesis, and decreasing gastrointestinal phosphate absorption [2] , [3] , [4] , [5] . Klotho-deficient mice have severe hyperphosphatemia due to defects in the Klotho-FGF23-vitamin D regulatory axis [5] , [6] , [7] . This phosphate retention is pivotal for growth retardation and premature death of Klotho-deficient mice. Dietary phosphate restriction rescues growth defects and premature death of the mice [5] , [6] , [7] . The notion that FGF receptor and Klotho form obligatory co-receptors for FGF23 is supported by the demonstration that systemic injection of bioactive FGF23 decreases serum levels of phosphate in wild–type (WT) mice, but not in Klotho-deficient mice [8] . The extracellular domain of Klotho is composed of two internal repeats, KL1 and KL2, each sharing amino-acid sequence homology to family 1 glycosidases [1] . The extracellular domain of Klotho is shed into the systemic circulation, urine and cerebrospinal fluid [9] . In urine, soluble Klotho regulates several ion transporters in the apical membrane of kidney tubules [10] , [11] , [12] . The physiological function of soluble Klotho present in the systemic circulation is mostly unknown. The heart responds to injury and stress signals by pathological growth and remodelling that often progresses to heart failure and sudden death [13] . One key regulatory step in the development of pathological cardiac growth and remodelling is activation of calmodulin-dependent serine–threonine protein phosphatase calcineurin by abnormal calcium signalling [14] . Once activated by increases in intracellular calcium, calcineurin dephosphorylates and causes nuclear translocation of nuclear factor of activated T cells (NFAT) transcription factors, which bind the regulator regions of cardiac genes and in conjunction with other transcription factors induce gene expression and promote hypertrophic growth and remodelling. Extracellular stimuli increase intracellular Ca 2+ levels by either promoting its release from intracellular organelles or its entry across the plasma membrane. The TRPC family channels are Ca 2+ -permeable cation channels expressed in the plasma membrane of many tissues including the heart [15] . The TRPC family includes seven members, and is divided into two groups based on structural and functional similarities: TRPC1/4/5, which are not sensitive to diacylglycerol (DAG), and TRPC3/6/7, which are activated by DAG. TRPC2 is not expressed in humans. Evidence indicates that Ca 2+ influx through cardiac TRPC channels—including TRPC1, 3, 4, 5 and 6—is important in calcineurin signalling and hypertrophic growth of hearts [16] , [17] , [18] , [19] , [20] , [21] , [22] . The expression of TRPC1, 3, 4, 5 and/or 6 is increased in hypertrophic hearts stimulated by various types or forms of stresses and their downregulation protects against cardiac hypertrophy. Some members of TRPC family channels, such as TRPC6, contain NFAT-responsive elements in their promoters, which have a pivotal role in amplifying and sustaining gene expression through a feed-forward circuit [16] . Thus, TRPC6 is an important modulator of cardiac hypertrophy and a potential target for treatment. However, physiological function of TRPC6 in the heart and its regulation remain poorly understood, limiting therapeutic strategies for targeting the pathway. Here we show that soluble Klotho inhibits cardiac TRPC6 channels and protects the heart against stress-induced pathological hypertrophy and remodelling. Klotho deficiency aggravates pathological heart growth Klotho expression is decreased in aging, a condition associated with increased risk for heart failure [23] , [24] . We examined the role of Klotho in protecting the heart using Klotho -hypomorphic mice rescued by dietary phosphate restriction. To avoid potential variations caused by strain and gender differences, we studied male mice congenic for the 129/SvJ background by backcrossing for >6 generations. As reported previously [5] , [6] , [7] , dietary phosphate restriction lowered serum phosphate levels and rescued growth defects and premature death of Klotho-deficient mice ( Supplementary Figs S1 and S2a ). Serum levels of sodium, potassium, chloride, calcium, magnesium and urea nitrogen were not different between WT and kl / kl mice on a phosphate-restricted diet ( Supplementary Table S1 ). Phosphate restriction did not affect the growth of WT mice ( Supplementary Fig. S1 ). Klotho -hypomorphic mice on low-phosphate diet remained markedly Klotho-deficient ( Supplementary Fig. S2b ). To investigate the potential cardioprotective effect of Klotho, we measured heart weight indices (heart weight normalized to body weight or tibia length) as well as the overall heart size in WT and Klotho-deficient mice. Heart weight indices ( Fig. 1a ) and the overall heart size measured using magnetic resonance imaging (MRI) ( Fig. 1c ) were not different between WT and Klotho-deficient mice at baseline. Overstimulation by isoproterenol (ISO) induced pathological hypertrophy in WT mice as reflected by increase in heart weight indices and the overall heart size, and these ISO-induced changes were aggravated in Klotho-deficient mice ( Fig. 1a–c ). ISO overstimulation is a well-accepted experimental model of stress-induced cardiac hypertrophy [25] , [26] . Phosphate restriction itself did not alter cardiac responses to stress, as baseline and ISO-induced increases in heart mass were not different between WT mice fed normal and phosphate-restricted diets ( Supplementary Fig. S2c ). 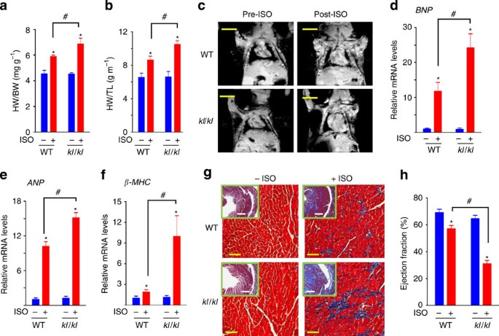Figure 1: Klotho-deficient mice display exaggerated ISO-induced cardiac hypertrophy. (a,b) Heart weight/body weight (HW/BW) (a) and heart weight/tibia length (HW/TL) (b) ratios of WT and homozygousklotho-hypomorphic mice (kl/kl) treated with ISO or vehicle (PBS). Mice were fed a low-phosphate diet after weaning. At the time of study (~3 months of age), body weight of WT andkl/klmice were not different (25.1±0.76 g versus 24.2±1.22 g). Also, systemic blood pressure of WT andkl/klmice were not different (systolic BP: 122±4 mm Hg versus 119±5 mm Hg). Data were mean±s.e.m.;n=6 for each group. *P<0.01 versus no ISO;#P<0.02 between indicated groups. (c) Magnetic resonance images of WT (n=5) andkl/kl(n=4) mice (along the long axis of hearts) before and after ISO treatment. Scale bar, 1 cm. (d–f) Expression ofANP(d),BNP(e) andβ-MHC(f) in hearts of WT andkl/klmice described ina, measured by quantitative RT–PCR, and normalized toGAPDH. Shown are mRNA levels relative to WT mice without ISO treatment (which is assigned the value 1). Data were mean±s.e.m.;n=6 for each group. *P<0.01 versus no ISO;#P<0.01 between indicated groups. (g) Heart sections of mice (a) were stained with Masson’s trichrome (blue is collagen). Magnification was × 200 and × 25 (insets), respectively. Yellow scale bar, 50 μm; white scale bar, 250 μm. (h) Ejection fraction of WT andkl/klmice (a) calculated based on left ventricular stroke and end-diastolic volumes measured by MRI (seeSupplementary Fig. S4for measurements). *P<0.01 versus no ISO;#P<0.01 between indicated groups. Figure 1: Klotho-deficient mice display exaggerated ISO-induced cardiac hypertrophy. ( a , b ) Heart weight/body weight (HW/BW) ( a ) and heart weight/tibia length (HW/TL) ( b ) ratios of WT and homozygous klotho -hypomorphic mice ( kl / kl ) treated with ISO or vehicle (PBS). Mice were fed a low-phosphate diet after weaning. At the time of study (~3 months of age), body weight of WT and kl / kl mice were not different (25.1±0.76 g versus 24.2±1.22 g). Also, systemic blood pressure of WT and kl / kl mice were not different (systolic BP: 122±4 mm Hg versus 119±5 mm Hg). Data were mean±s.e.m. ; n =6 for each group. * P <0.01 versus no ISO; # P <0.02 between indicated groups. ( c ) Magnetic resonance images of WT ( n =5) and kl / kl ( n =4) mice (along the long axis of hearts) before and after ISO treatment. Scale bar, 1 cm. ( d – f ) Expression of ANP ( d ), BNP ( e ) and β-MHC ( f ) in hearts of WT and kl / kl mice described in a , measured by quantitative RT–PCR, and normalized to GAPDH . Shown are mRNA levels relative to WT mice without ISO treatment (which is assigned the value 1). Data were mean±s.e.m. ; n =6 for each group. * P <0.01 versus no ISO; # P <0.01 between indicated groups. ( g ) Heart sections of mice ( a ) were stained with Masson’s trichrome (blue is collagen). Magnification was × 200 and × 25 (insets), respectively. Yellow scale bar, 50 μm; white scale bar, 250 μm. ( h ) Ejection fraction of WT and kl / kl mice ( a ) calculated based on left ventricular stroke and end-diastolic volumes measured by MRI (see Supplementary Fig. S4 for measurements). * P <0.01 versus no ISO; # P <0.01 between indicated groups. Full size image Pathological cardiac hypertrophy and remodelling are also characterized by increased (re)expression of fetal genes that are normally quiescent in adult hearts, including brain natriuretic peptide ( BNP ), atrial natriuretic peptide ( ANP ) and β-myosin heavy chain ( β - MHC ) [13] , [14] . Consistent with the notion that Klotho deficiency accelerates ISO-induced pathological cardiac remodelling, the expression of cardiac fetal genes was increased by ISO in WT mice, and such increase in gene expression was augmented in Klotho-deficient mice ( Fig.1d–f ). Increased expression of these cardiac fetal genes is mediated by activation of the calcineurin-NFAT pathway [14] . The Trpc6 gene contains NFAT-responsive elements in the promoter and its expression is upregulated in several human and rodent models of heart failure [16] , [17] , [20] . We therefore measured the expression of Trpc6 in ISO-treated WT and Klotho-deficient hearts. Trpc6 mRNA levels were increased in WT hearts after ISO treatment ( Supplementary Fig. S3a ). For comparison, ISO treatment did not alter the expression of Trpc6 in other tissues including the blood vessels, lung, kidney and liver. As was observed for cardiac fetal genes, ISO-induced increases in Trpc6 mRNA were enhanced in Klotho-deficient relative to WT mice ( Supplementary Fig. S3b ). Interstitial fibrosis is another consequence of pathological cardiac hypertrophy and remodelling [16] . Trichrome staining of heart sections revealed fibrosis in WT hearts after ISO treatment, and Klotho deficiency worsened ISO-induced cardiac fibrosis ( Fig. 1g ). In support of these results from morphometric and gene expression studies, functional analysis of hearts using MRI showed that ISO treatment decreased the ejection fraction of WT hearts, and Klotho-deficiency markedly aggravated the ISO-induced decline in the ejection fraction ( Fig. 1h ). Left ventricular end-systolic and end-diastolic volumes were markedly increased, and stroke volumes were decreased in Klotho-deficient mice after ISO treatment ( Supplementary Fig. S4a ,b), indicating chamber dilatation as well as impaired contractility of the left ventricle (LV). Severe heart failure with lung oedema developed in some Klotho-deficient mice after ISO treatment ( Supplementary Fig. S4c,d ). Thus, Klotho deficiency does not cause baseline cardiac abnormalities but renders the heart more susceptible to stress-induced pathological cardiac remodelling. Klotho attenuates stress-induced cardiac hypertrophy To further corroborate the above experimental data indicating that Klotho protects the heart against stress-induced cardiac remodelling, we examined ISO-induced cardiac changes in transgenic mice that overexpress Klotho (KL-Tg). These mice live ~20–30% longer than WT littermates, and the circulating level of soluble Klotho in transgenic mice is ~100% higher than WT (~200 pM in transgenic mice versus ~100 pM in WT mice) [27] . Klotho overexpression in mice did not cause detectable changes in heart mass index and the heart size at baseline ( Fig. 2a ), and nor did it alter the systemic blood pressure (systolic BP: 103±7 mm Hg and 103±4 mm Hg, WT versus KL-Tg, n =4 each). Klotho overexpression yet blunted the ISO-induced cardiac hypertrophic responses ( Fig. 2a ). Consistent with the notion that Klotho protects against stress-induced cardiac remodelling, Klotho overexpression did not alter BNP and Trpc6 mRNA levels at baseline, but attenuated ISO-induced increases in BNP and Trpc6 mRNA expression ( Fig. 2c ). It has been reported that elevated serum FGF23 promotes cardiac hypertrophy [28] . Because Klotho and FGF23 work in the same pathway to regulate phosphate metabolism, we measured serum phosphate and FGF23 levels. Klotho overexpression in mice did not alter serum phosphate or FGF23 levels ( Fig. 2e ), indicating that the cardioprotective effect of Klotho was not mediated by serum FGF23. As Klotho overexpression mice and control WT littermates were fed normal phosphate diets, these studies also exclude the role of dietary phosphate restriction in cardioprotection by Klotho. 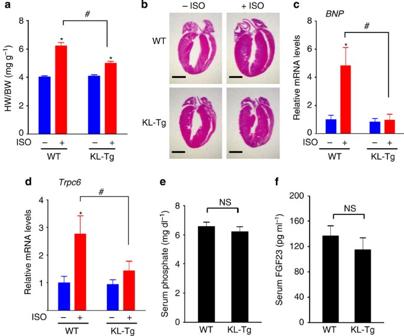Figure 2: Klotho overexpression in mice attenuates cardiac hypertrophic responses to ISO. (a) Heart weight/body weight (HW/BW) ratios of WT and KL-Tg±ISO treatment (n=8 each). Mice were fed a normal phosphate diet after weaning, and studied at 3 months of age. *P<0.01 versus no ISO;#P<0.02 between indicated groups. (b) Representative haematoxylin and eosin-stained heart sections of WT and KL-Tg mice described ina. Scale bar, 2 mm. (c,d) The expression ofBNP(c) andTrpc6(d) in hearts of WT and KL-Tg mice described above.n=8 each group. *P<0.01 versus no ISO;#P<0.02 between indicated groups. (e,f) Serum phosphate (e) and FGF23 (f) levels of WT and KL-Tg mice before ISO treatment.n=8 each. ns, not significant. All data are expressed as mean±s.e.m. Figure 2: Klotho overexpression in mice attenuates cardiac hypertrophic responses to ISO. ( a ) Heart weight/body weight (HW/BW) ratios of WT and KL-Tg±ISO treatment ( n =8 each). Mice were fed a normal phosphate diet after weaning, and studied at 3 months of age. * P <0.01 versus no ISO; # P <0.02 between indicated groups. ( b ) Representative haematoxylin and eosin-stained heart sections of WT and KL-Tg mice described in a . Scale bar, 2 mm. ( c , d ) The expression of BNP ( c ) and Trpc6 ( d ) in hearts of WT and KL-Tg mice described above. n =8 each group. * P <0.01 versus no ISO; # P <0.02 between indicated groups. ( e , f ) Serum phosphate ( e ) and FGF23 ( f ) levels of WT and KL-Tg mice before ISO treatment. n =8 each. ns, not significant. All data are expressed as mean±s.e.m. Full size image Klotho protects the heart by downregulation of TRPC6 Next, we investigated the mechanism by which Klotho protects against stress-induced cardiac hypertrophy and remodelling. We have observed that Klotho-deficiency aggravated ISO-induced increases in Trpc6 expression, and conversely Klotho overexpression attenuated the ISO-induced increases in cardiac Trpc6 mRNA expression ( Supplementary Fig. S3b and Fig. 2d ). Inhibition of cardiac TRPC6 by gene silencing or by dominant-negative expression of mutant channels confers cardioprotection [17] , [20] . We examined whether Klotho may protect the heart by inhibiting TRPC6 by crossing Klotho-deficient mice with global Trpc6 -knockout mice [29] . Mice with global deletion of Trpc6 grow normally and have no apparent defects in major organ systems at baseline [30] . Consistently, we found that the baseline heart mass index was not different between mice with global deletion of Trpc6 and control WT littermates ( Fig. 3a ). Deletion of Trpc6 partially protected against ISO-induced cardiac remodelling, but completely prevented the exaggerated ISO-induced cardiac hypertrophy in Klotho-deficient mice. Consistent with these results, deletion of Trpc6 attenuated ISO-induced increases in ANP and BNP mRNA, and abolished the exaggerated ISO-induced increases in the mRNA in Klotho-deficient mice ( Fig. 3b ). 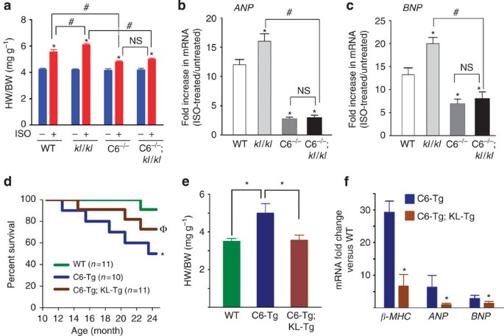Figure 3: Klotho and TPRC6 exert opposite effects on cardiac hypertrophy. (a) Heart weight/body weight (HW/BW) ratios of WT,kl/kl, homozygousTrpc6-knockout (C6−/−) and C6−/−;kl/kldouble-mutant mice±ISO treatment. All mice were fed a low-Pi diet after weaning and ~3 months of age (n=6–8 for each group). *P<0.01 versus no ISO;#P<0.02 between indicated groups. (b,c) ISO-induced increases of expression ofANP(b) andBNP(c) in hearts of above mice. Abundance of mRNA determined by real-time RT–PCR was plotted as fold increase in ISO-treated group versus sham (ISO-untreated) group.n=6–8 for each group. *P<0.01 versus WT;#P<0.01 between indicated groups. (d) Kaplan–Meier survival analysis of WT, cardiac-specific TRPC6-overexpressing transgenic mice (C6-Tg) and double-transgenic mice (C6-Tg; KL-Tg) mice at ~24 months.n=5 each group. *P<0.01 versus WT; Ф, not significant versus either WT or C6-Tg. (e) HW/BW ratios of WT, C6-Tg and C6-Tg; KL-Tg living mice at ~24 months.n=5 each group. *P<0.01 between indicated groups. (f) Changes ofβ-MHC,ANPandBNPexpression in hearts of C6-Tg and double Tg mice versus WT mice. mRNA abundance in the hearts of the groups inewere plotted as fold changes versus WT group.n=5 each group. *P<0.01 versus C6-Tg. Data ina–c,e–fare expressed as mean±s.e.m. Figure 3: Klotho and TPRC6 exert opposite effects on cardiac hypertrophy. ( a ) Heart weight/body weight (HW/BW) ratios of WT, kl / kl , homozygous Trpc6 -knockout (C6 −/− ) and C6 −/− ; kl / kl double-mutant mice±ISO treatment. All mice were fed a low-Pi diet after weaning and ~3 months of age ( n =6–8 for each group). * P <0.01 versus no ISO; # P <0.02 between indicated groups. ( b , c ) ISO-induced increases of expression of ANP ( b ) and BNP ( c ) in hearts of above mice. Abundance of mRNA determined by real-time RT–PCR was plotted as fold increase in ISO-treated group versus sham (ISO-untreated) group. n =6–8 for each group. * P <0.01 versus WT; # P <0.01 between indicated groups. ( d ) Kaplan–Meier survival analysis of WT, cardiac-specific TRPC6-overexpressing transgenic mice (C6-Tg) and double-transgenic mice (C6-Tg; KL-Tg) mice at ~24 months. n =5 each group. * P <0.01 versus WT; Ф, not significant versus either WT or C6-Tg. ( e ) HW/BW ratios of WT, C6-Tg and C6-Tg; KL-Tg living mice at ~24 months. n =5 each group. * P <0.01 between indicated groups. ( f ) Changes of β-MHC , ANP and BNP expression in hearts of C6-Tg and double Tg mice versus WT mice. mRNA abundance in the hearts of the groups in e were plotted as fold changes versus WT group. n =5 each group. * P <0.01 versus C6-Tg. Data in a – c , e – f are expressed as mean±s.e.m. Full size image We further investigated cardioprotection by Klotho using transgenic mice that overexpress TRPC6 in hearts. Mice with cardiac-specific overexpression of TRPC6 develop spontaneous cardiac hypertrophy and also have heightened sensitivity to stress-induced hypertrophy [16] . We crossed mice with cardiac TRPC6 overexpression with transgenic mice overexpressing Klotho to create double transgenic mice, and compared the survival rate, heart mass index and cardiac fetal gene expression of double transgenic mice with those having cardiac overexpression of TRPC6 and with WT littermates. Compared with WT littermates at 24 months of age, cardiac TRPC6-overexpressing mice had decreased survival and increased heart mass index and cardiac fetal gene expression without ISO treatment ( Fig. 3d–f ). Klotho overexpression tended to improve the survival of cardiac TRPC6-overexpressing mice, prevented the increase in heart mass, and markedly diminished the increase in fetal gene expression induced by overexpression of TRPC6 in hearts. These studies also support the notion that Klotho protects the heart by inhibiting cardiac TRPC6. Soluble Klotho inhibits TRPC6 in isolated cardiac myocytes Klotho is not expressed in the heart. We tested the hypothesis that soluble Klotho present in the systemic circulation mediates the inhibition of cardiac TRPC6. TRPC6 is activated by DAG [15] . We examined TRPC6 channel activity in freshly isolated ventricular myocytes by whole-cell patch-clamp recording using stimulation by endothelin-1 (ET1) to release DAG ( Fig. 4a ). Ventricular myocytes from WT mice without ISO treatment showed baseline ET-1-activated TRPC-like currents presumably mediated by non-TRPC6 channels, as currents were not different between Trpc6 -knockout mice (C6 −/− ) and WT littermates ( Fig. 4b ). ISO treatment increased TRPC6-mediated currents in WT hearts ( Fig. 4a ); the role of TRPC6 is supported by the facts that the increase was eliminated in Trpc6 -knockout mice ( Fig. 4b ), and identical currents were seen in TRPC6-overexpressing hearts ( Fig. 4a and Supplementary Fig. S5 ). Cell capacitance (a measurement of surface area of cells) of ventricular myocytes was increased in WT hearts after ISO and in TRPC6-overexpressing hearts ( Fig. 4c ), supporting the conclusion that myocyte hypertrophy occurred under these conditions. Klotho overexpression in mice prevented the ISO-induced increases in currents ( Fig. 4b ), and acute addition of soluble Klotho to culture media decreased TRPC6-mediated currents in myocytes isolated from WT mice after ISO treatment ( Fig. 4d ). Similarly, direct addition of soluble Klotho inhibited the currents in myocytes isolated from TRPC6-overexpressing mice ( Fig. 4e ). It is theoretically possible that Klotho inhibits TRPC6 by decreasing the production of DAG. However, soluble Klotho decreased TRPC6 currents in cardiomyocytes directly activated by membrane-permeant DAG ( Fig. 4f ), indicating that it inhibits cardiac TRPC6 channel function acting downstream of DAG. 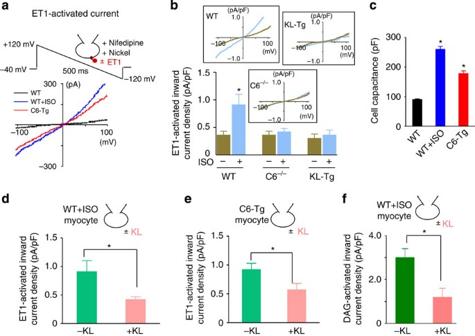Figure 4: Soluble Klotho inhibits TRPC6 currents in isolated ventricular myocytes. (a) Top panel shows recording conditions. Currents were recorded in ruptured whole-cell mode. Voltage protocol consists of holding at −40 mV and repetitive descending ramp pulses (500 ms duration) from +120 to −120 mV. This protocol diminishes the activation of Nav. Bath solution contains inhibitors for L-type Cavchannel (Nifedipine, 1 μM) and Na+–Ca2+exchanger (NiCl2, 3 mM). Bottom panel shows representative current–voltage (I–V) relationships of currents activated by ET1 (20 nM) in myocytes isolated from WT mice, WT mice after ISO treatment, and from C6-Tg mice.n=7–9 each group. (b) Currents were recorded from myocytes isolated from WT, C6−/−and KL-Tg mice treated with or without ISO. Inward current density (current at −100 mV divided by cell capacitance; pA/pF) is shown.n=7–9 for each group. *P<0.01 versus no ISO. (c) Cell capacitance of myocytes recorded described ina.n=7–9 for each group. (d) Myocytes were isolated from WT mice treated with ISO and incubated with or without purified recombinant soluble Klotho (200 pM for 2 h) before ruptured whole-cell recording.n=6 each. *P<0.01 versus no KL. (e) Myocytes were isolated from C6-Tg mice and incubated with or without purified recombinant soluble Klotho before ruptured whole-cell recording.n=7 each. *P<0.01 versus no KL. (f) Myocytes were isolated from WT mice treated with ISO and incubated with or without purified recombinant soluble Klotho before ruptured whole-cell recording. TRPC6 currents were activated by extracellular addition of a membrane-permeant DAG (1-oleoyl-2-acetyl glycerol, 50 μM). Activation of TRPC6 occurred within 1–2 min.n=8 each. *P<0.01 versus no KL. Data inb–fare expressed as mean±s.e.m. Figure 4: Soluble Klotho inhibits TRPC6 currents in isolated ventricular myocytes. ( a ) Top panel shows recording conditions. Currents were recorded in ruptured whole-cell mode. Voltage protocol consists of holding at −40 mV and repetitive descending ramp pulses (500 ms duration) from +120 to −120 mV. This protocol diminishes the activation of Na v . Bath solution contains inhibitors for L-type Ca v channel (Nifedipine, 1 μM) and Na + –Ca 2+ exchanger (NiCl 2 , 3 mM). Bottom panel shows representative current–voltage (I–V) relationships of currents activated by ET1 (20 nM) in myocytes isolated from WT mice, WT mice after ISO treatment, and from C6-Tg mice. n =7–9 each group. ( b ) Currents were recorded from myocytes isolated from WT, C6 −/− and KL-Tg mice treated with or without ISO. Inward current density (current at −100 mV divided by cell capacitance; pA/pF) is shown. n =7–9 for each group. * P <0.01 versus no ISO. ( c ) Cell capacitance of myocytes recorded described in a . n =7–9 for each group. ( d ) Myocytes were isolated from WT mice treated with ISO and incubated with or without purified recombinant soluble Klotho (200 pM for 2 h) before ruptured whole-cell recording. n =6 each. * P <0.01 versus no KL. ( e ) Myocytes were isolated from C6-Tg mice and incubated with or without purified recombinant soluble Klotho before ruptured whole-cell recording. n =7 each. * P <0.01 versus no KL. ( f ) Myocytes were isolated from WT mice treated with ISO and incubated with or without purified recombinant soluble Klotho before ruptured whole-cell recording. TRPC6 currents were activated by extracellular addition of a membrane-permeant DAG (1-oleoyl-2-acetyl glycerol, 50 μM). Activation of TRPC6 occurred within 1–2 min. n =8 each. * P <0.01 versus no KL. Data in b – f are expressed as mean±s.e.m. Full size image Klotho blocks IGF and PI3K-dependent exocytosis of TRPC6 Because isolated mouse cardiomyocytes cannot be cultured continuously and the low abundance of endogenous TRPC6 in hearts, we further investigated the mechanism of regulation by soluble Klotho using HEK cells expressing recombinant TRPC6 as well as isolated cardiac myocytes. As in cardiomyocytes, soluble Klotho decreased DAG-activated TRPC6 channels in HEK cells ( Fig. 5a ). Soluble Klotho treatment decreased cell surface abundance of TRPC6 measured by biotinylation assays ( Fig. 5b ). Soluble Klotho exhibits sialidase (Sial) activity and increases cell surface abundance of TRPV5 channels by cleaving sialic acids in the N-glycans of channels [11] . The Sial activity of Klotho is not responsible for the regulation of TRPC6, as purified Sial had no effect on TRPC6 whereas it stimulated TRPV5 ( Fig. 5c ). The above results also indicate that soluble Klotho decreases cell surface expression of TRPC6 via a mechanism not restricted to cardiomyocytes. 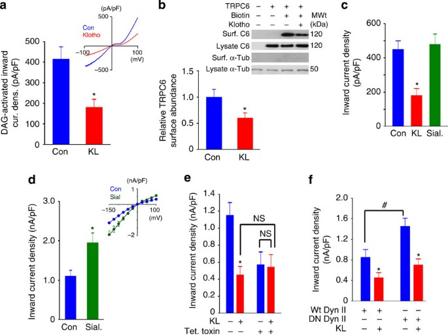Figure 5: Soluble Klotho (sKlotho) decreases cell surface abundance of TRPC6. (a) sKlotho inhibits recombinant TRPC6 channels. HEK cells expressing HA-tagged TRPC6 were incubated with or without purified recombinant soluble Klotho11,27(KL 200 pM for 2 h) before ruptured whole-cell recording. TRPC6 currents were activated by membrane-permeant DAG. Shown is inward current density at −100 mV (n=7 for each). *P<0.01 versus control (no KL). In control cells without expression of recombinant TRPC6, inward current density after application of DAG was 21±5 pA/pF (at −100 mV;n=9). Note that I–V curves for recombinant TRPC6 currents shown here are more strongly double-rectifying than for native currents shown inFigure 4a. The differences may be partly due to formation of heteromultimers of TRPC6 with other TRPC members in native hearts. (b) Soluble Klotho decreases TRPC6 cell surface (labelled as ‘Surf’) abundance. Specific biotinylation of membrane TRPC6 was supported by lack of detection of α-tubulin in the membrane fraction. The abundance of α-tubulin (labelled as ‘α-Tub’) in lysates served as a loading control. Bar graph shows mean±s.e.m. of four separate experiments. TRPC6 bands (detected by anti-HA antibody) were quantified by densitometry. *P<0.05 versus control (no KL). (c) Soluble Klotho, but not purified sialidase11(Sial, 0.3 U ml−1), inhibits TRPC6.n=6 for each. *P<0.01 versus control (no KL). (d) Purified Sial increases TRPV5 currents. Whole-cell TRPV5 currents were recorded as described11.n=6 each. (e) Tetanus (tet.) toxin decreases TRPC6 currents, and prevent the inhibition by soluble Klotho. TRPC6-expressing cells were preincubated with tetanus toxin (50 nM for 3 h) before soluble Klotho.n=6–7 for each. *P<0.01 versus control (no KL). ns, not significant between indicated groups. (f) Role of endocytosis in inhibition of TRPC6 by Klotho. TRPC6 was coexpressed with a dominant-negative (K44A; lysine-44 to alanine mutation; DN Dyn II) or WT dynamin II (Wt DN II).n=7–8 for each. *P<0.01 versus control (no KL).#P<0.02 between indicated groups. All data are expressed as mean±s.e.m. Con, control; Sial., sialidase; surf., surface; Tet., tetanus. Figure 5: Soluble Klotho (sKlotho) decreases cell surface abundance of TRPC6. ( a ) sKlotho inhibits recombinant TRPC6 channels. HEK cells expressing HA-tagged TRPC6 were incubated with or without purified recombinant soluble Klotho [11] , [27] (KL 200 pM for 2 h) before ruptured whole-cell recording. TRPC6 currents were activated by membrane-permeant DAG. Shown is inward current density at −100 mV ( n =7 for each). * P <0.01 versus control (no KL). In control cells without expression of recombinant TRPC6, inward current density after application of DAG was 21±5 pA/pF (at −100 mV; n =9). Note that I–V curves for recombinant TRPC6 currents shown here are more strongly double-rectifying than for native currents shown in Figure 4a . The differences may be partly due to formation of heteromultimers of TRPC6 with other TRPC members in native hearts. ( b ) Soluble Klotho decreases TRPC6 cell surface (labelled as ‘Surf’) abundance. Specific biotinylation of membrane TRPC6 was supported by lack of detection of α-tubulin in the membrane fraction. The abundance of α-tubulin (labelled as ‘α-Tub’) in lysates served as a loading control. Bar graph shows mean±s.e.m. of four separate experiments. TRPC6 bands (detected by anti-HA antibody) were quantified by densitometry. * P <0.05 versus control (no KL). ( c ) Soluble Klotho, but not purified sialidase [11] (Sial, 0.3 U ml −1 ), inhibits TRPC6. n =6 for each. * P <0.01 versus control (no KL). ( d ) Purified Sial increases TRPV5 currents. Whole-cell TRPV5 currents were recorded as described [11] . n =6 each. ( e ) Tetanus (tet.) toxin decreases TRPC6 currents, and prevent the inhibition by soluble Klotho. TRPC6-expressing cells were preincubated with tetanus toxin (50 nM for 3 h) before soluble Klotho. n =6–7 for each. * P <0.01 versus control (no KL). ns, not significant between indicated groups. ( f ) Role of endocytosis in inhibition of TRPC6 by Klotho. TRPC6 was coexpressed with a dominant-negative (K44A; lysine-44 to alanine mutation; DN Dyn II) or WT dynamin II (Wt DN II). n =7–8 for each. * P <0.01 versus control (no KL). # P <0.02 between indicated groups. All data are expressed as mean±s.e.m. Con, control; Sial., sialidase; surf., surface; Tet., tetanus. Full size image The decrease in cell-surface abundance of TRPC6 by soluble Klotho may be caused by decreased exocytosis and/or increased endocytosis of the channel. Blocking exocytosis by v-SNARE inhibitor tetanus toxin [31] decreased TRPC6 currents, and prevented further inhibition by soluble Klotho ( Fig. 5e ). Because tetanus toxin completely prevented the effect by Klotho, the major (if not the sole) action of Klotho on TRPC6 is by blocking exocytosis. Consistent with this notion, we found that blocking endocytosis using a dominant-negative dynamin did not affect the ability of Klotho to inhibit TRPC6: Coexpression with dominant-negative dynamin increased the basal (that is, without KL) TRPC6 currents, indicating inhibition of endocytosis of channels, but soluble Klotho decreased TRPC6 currents similarly in cells expressing dominant-negative dynamin and in cell expressing the control WT dynamin ( Fig. 5f ). Phosphoinositide-3-kinase (PI3K)-activating growth factors increase cell surface abundance of TRPC channels by stimulating exocytosis [32] . Soluble Klotho inhibits PI3K signalling by insulin and insulin-like growth factors (IGF), which contributes to the antiaging and tumor suppression effects of Klotho [27] , [33] , [34] , [35] . We therefore tested the hypothesis that soluble Klotho inhibits TRPC6 by interfering with IGF1 activation of PI3K to promote exocytosis of channels. To allow for studying the effect of IGF1, we first examined the effect of serum deprivation. Serum deprivation lowered TRPC6 cell surface abundance and activities, and prevented the inhibition by soluble Klotho ( Fig. 6a ). The role of IGF1 is demonstrated by findings showing that physiological concentrations of IGF1 (10 nM) reproduced the effect of serum to promote TRPC6 currents and that soluble Klotho inhibited IGF1-stimulated TRPC6 currents ( Fig. 6c ). Moreover, PI3K inhibitor wortmannin decreased TRPC6 currents stimulated by IGF1, and prevented a further decrease of TRPC6 by soluble Klotho ( Fig. 6d ). These results support the notion that soluble Klotho inhibits IGF1 and PI3K-dependent exocytosis of TRPC6. Because wortmannin abrogates its effect, soluble Klotho acts upstream of PI3K. 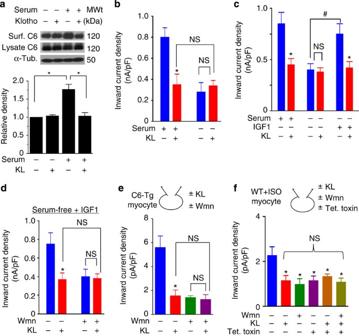Figure 6: Soluble Klotho inhibits TRPC6 by blocking PI3K-dependent channel exocytosis. (a) Effect of serum deprivation on TRPC6 cell surface abundance and the regulation by soluble Klotho. HEK cells expressing TRPC6 were cultured in serum-deprived or serum-containing media for 24 h and further incubated with soluble Klotho (200 pM) for 2 h before subjecting to biotinylation assay. The abundance of α-tubulin in lysates served as a loading control. Bar graph shows mean±s.e.m. of four separate experiments. *P<0.05 between indicated groups. (b) DAG-stimulated TRPC6 current density in HEK cells cultured in serum-deprived or serum-containing media and incubated with or without soluble Klotho for 2 h.n=6–9 for each. *P<0.01 versus no KL. ns, not significant between indicated groups. (c) HEK cells were cultured in serum-containing or serum-free medium with or without IGF1 (10 nM) for 24 h, and incubated with or without soluble Klotho for 2 h before recording.n=7–9 for each. *P<0.01 versus no KL.#P<0.01 between indicated groups. (d) HEK cells cultured with IGF1 in the serum-free medium for 24 h were preincubated with PI3K inhibitor wortmannin (Wmn; 50 nM) or vehicle (dimethylsulphoxide) for 2 h and further incubated with or without soluble Klotho for 2 h before recording.n=8–9 for each. *P<0.01 versus no KL. ns, not significant between indicated groups. (e) Cardiomyocytes isolated from C6-Tg mice were preincubated with wortmannin (50 nM) or vehicle for 2 h and further incubated with or without soluble Klotho for 2 h before recording. Shown is ET1-activated TRPC6 current density (pA/pF at −100 mV).n=8–10 for each. *P<0.01 versus no KL. ns, not significant between indicated groups. Note that cardiomyocytes were maintained in a serum-free solution after isolation, and that PI3K signalling cascade apparently remained active during our experiments (within 4 h of isolation). (f) No additive effects between inhibition of TRPC6 by tetanus (Tet.) toxin, by wortmannin and by soluble Klotho in cardiomyocytes from WT mice after ISO treatment. *P<0.01 versus control; ns, not significant between each two groups. All data are expressed as mean±s.e.m. Surf., surface. Figure 6: Soluble Klotho inhibits TRPC6 by blocking PI3K-dependent channel exocytosis. ( a ) Effect of serum deprivation on TRPC6 cell surface abundance and the regulation by soluble Klotho. HEK cells expressing TRPC6 were cultured in serum-deprived or serum-containing media for 24 h and further incubated with soluble Klotho (200 pM) for 2 h before subjecting to biotinylation assay. The abundance of α-tubulin in lysates served as a loading control. Bar graph shows mean±s.e.m. of four separate experiments. * P <0.05 between indicated groups. ( b ) DAG-stimulated TRPC6 current density in HEK cells cultured in serum-deprived or serum-containing media and incubated with or without soluble Klotho for 2 h. n =6–9 for each. * P <0.01 versus no KL. ns, not significant between indicated groups. ( c ) HEK cells were cultured in serum-containing or serum-free medium with or without IGF1 (10 nM) for 24 h, and incubated with or without soluble Klotho for 2 h before recording. n =7–9 for each. * P <0.01 versus no KL. # P <0.01 between indicated groups. ( d ) HEK cells cultured with IGF1 in the serum-free medium for 24 h were preincubated with PI3K inhibitor wortmannin (Wmn; 50 nM) or vehicle (dimethylsulphoxide) for 2 h and further incubated with or without soluble Klotho for 2 h before recording. n =8–9 for each. * P <0.01 versus no KL. ns, not significant between indicated groups. ( e ) Cardiomyocytes isolated from C6-Tg mice were preincubated with wortmannin (50 nM) or vehicle for 2 h and further incubated with or without soluble Klotho for 2 h before recording. Shown is ET1-activated TRPC6 current density (pA/pF at −100 mV). n =8–10 for each. * P <0.01 versus no KL. ns, not significant between indicated groups. Note that cardiomyocytes were maintained in a serum-free solution after isolation, and that PI3K signalling cascade apparently remained active during our experiments (within 4 h of isolation). ( f ) No additive effects between inhibition of TRPC6 by tetanus (Tet.) toxin, by wortmannin and by soluble Klotho in cardiomyocytes from WT mice after ISO treatment. * P <0.01 versus control; ns, not significant between each two groups. All data are expressed as mean±s.e.m. Surf., surface. Full size image Finally, we examined whether soluble Klotho regulates TRPC6 in hearts via the same mechanism. Wortmannin decreased TRPC6 currents and prevented the inhibition by soluble Klotho in isolated cardiomyocytes ( Fig. 6e ). Furthermore, the effect of wortmannin to decrease cardiac TRPC6 currents and to prevent further inhibition by soluble Klotho was reproduced by tetanus toxin, and the effects of wortmannin and tetanus toxin were not additive ( Fig. 6f ). Thus, tetanus toxin and wortmannin inhibit cardiac TRPC6 via the same mechanism; that is, by blocking exocytosis of channels. Collectively, these data strongly support the hypothesis that soluble Klotho inhibits TRPC6 by blocking PI3K-dependent exocytosis of channels ( Fig. 7 ). 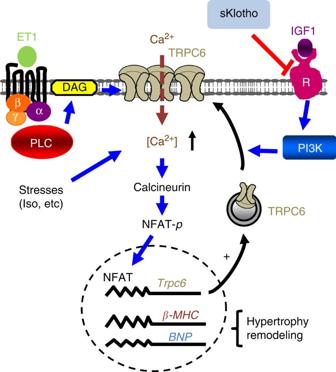Figure 7: Working model for Klotho-mediated inhibition of TRPC6. Normally, TRPC6 channel activity is undetectable in hearts. Stresses (such as ISO overstimulation in this study) cause an abnormal intracellular Ca2+signalling, which activates calcineurin and NFAT, thereby inducing cardiac hypertrophy and remodelling, as well asTrpc6gene expression. Upregulation of TRPC6 provides a feed-forward loop that amplifies and sustains the pathological cardiac responses. IGF1 activates PI3K to promote exocytosis of TRPC6. Soluble Klotho (sKlotho) inhibits IGF1 activation of PI3K, partly by direct interactions with the receptors. Inhibition of TRPC6 by sKlotho targeting at IGF1 and PI3K protects the heart from stress-induced cardiac hypertrophy. Without stress signal to upregulate TRPC6 expression, sKlotho has no effect on the heart at baseline. PLC, phospholipase C. Figure 7: Working model for Klotho-mediated inhibition of TRPC6. Normally, TRPC6 channel activity is undetectable in hearts. Stresses (such as ISO overstimulation in this study) cause an abnormal intracellular Ca 2+ signalling, which activates calcineurin and NFAT, thereby inducing cardiac hypertrophy and remodelling, as well as Trpc6 gene expression. Upregulation of TRPC6 provides a feed-forward loop that amplifies and sustains the pathological cardiac responses. IGF1 activates PI3K to promote exocytosis of TRPC6. Soluble Klotho (sKlotho) inhibits IGF1 activation of PI3K, partly by direct interactions with the receptors. Inhibition of TRPC6 by sKlotho targeting at IGF1 and PI3K protects the heart from stress-induced cardiac hypertrophy. Without stress signal to upregulate TRPC6 expression, sKlotho has no effect on the heart at baseline. PLC, phospholipase C. Full size image The data presented in this study provide compelling evidence indicating that soluble Klotho protects the heart against stress-induced cardiac hypertrophy and remodelling. Klotho expression is decreased in aging [23] , thus decline in circulating soluble Klotho may contribute to age-related cardiomyopathy in humans. One consequence of cardiac aging is increased sensitivity to stress-induced heart failure [36] similar to the changes in Klotho-deficient mice we observed here. Many Klotho-mediated aging phenotypes, such as vascular calcification, growth defects and premature death, are attributed to defects in the function of membrane Klotho as co-receptors for FGF23 and phosphate retention [3] , [4] , [5] , [6] , [7] , [8] . Our results indicate that the cardioprotective effect of soluble Klotho is independent of FGF23 and phosphate metabolism. First, Klotho overexpression in mice confers cardioprotection without altering serum phosphate and FGF23 levels. Second, dietary phosphate restriction normalizes serum phosphate levels of Klotho-deficient mice to the level of WT mice, excluding hyperphosphatemia as the culprit of cardiac dysfunction in these mice. Moreover, deletion of Trpc6 completely prevents exaggerated stress-induced cardiac hypertrophy and remodelling in Klotho-deficient mice, indicating that cardioprotection by Klotho is mediated by downregulation of TRPC6. TRPC6 is broadly expressed in tissues [15] , [37] . Although it is possible that the effect of Klotho on TRPC6 in other tissues also contributes to cardioprotection, the following results indicate that Klotho inhibition of cardiac TRPC6 has a critical role in the process. First, Klotho ameliorates cardiac hypertrophy and remodelling induced by heart-specific overexpression of TRPC6, and Klotho inhibits TRPC6 in isolated cardiomyocytes. Second, Klotho-deficient mice have no cardiac dysfunction at baseline, but develop exaggerated cardiomyopathy in response to ISO treatment. ISO treatment causes upregulation of Trpc6 mRNA in the heart, but not in other tissues that influence cardiac function, such as the blood vessels, lung, and kidney. The effect of Trpc6 deletion to prevent ISO-induced exaggerated cardiomyopathy in Klotho-deficient mice is therefore most likely due to abolition of ISO-induced increases of cardiac TRPC6. Our findings also have important implications in chronic kidney disease (CKD), a disease that affects ~10% of the general population [38] , [39] . The prevalence of cardiac hypertrophy in patients of advanced stages of CKD is estimated as high as 90%, and cardiac dysfunction is the main cause of death for the patients [39] , [40] , [41] . Klotho is predominantly produced in the kidney, and circulating levels of soluble Klotho are reportedly decreased in CKD [42] , [43] . Our study supports that decreased levels of soluble Klotho contribute to the pathogenesis of cardiac hypertrophy in CKD. Recently, Faul et al. reported that FGF23 stimulates cardiomyocyte growth and increased serum FGF23 contributes to cardiac hypertrophy in CKD [28] . Interestingly, FGF23 appears to induce cardiac hypertrophy independently of stress factors, whereas Klotho deficiency predisposes the heart to stress-induced pathological hypertrophy. Thus, increased FGF23 and Klotho deficiency may synergistically contribute to cardiac hypertrophy in CKD by participating at different stages of pathogenesis. The physiological role of TRPC6 in hearts is elusive. Its function appears to be dispensable, as mice with deletion of Trpc6 have no apparent cardiac dysfunction. Consistent with this observation, we found that TRPC6 channel activity is undetectable in hearts at baseline. Overstimulation by ISO leads to increase in Trpc6 mRNA levels and functional TRPC6 currents in mouse hearts. Increased expression of cardiac TRPC6 has also been reported in mouse models of cardiac hypertrophy induced by calcineurin gene overexpression, by overstimulation by neuroendocrine hormones including ET-1, phenylephrine and angiotensin II, by thoracic aortic banding pressure overload, and in human failing hearts [16] , [17] , [20] . Thus, soluble Klotho protects the heart by acting on a molecule that is normally quiescent but activated during stresses. Mechanistically, we propose that IGFs such as IGF1 provide a tonic stimulation for exocytosis of TRPC6 via PI3K, and soluble Klotho exerts a tonic inhibition to the system (model in Fig. 7 ). Cardiac stresses increase the intracellular Ca 2+ concentration from multiple mechanisms [44] . The abnormal intracellular calcium signalling in the heart activates calcineurin and NFAT to initiate fetal gene expression and pathological cardiac hypertrophy and remodelling. TRPC6 contains NFAT-responsive elements in its promoter and is also upregulated by stress. The increased Ca 2+ influx through TRPC6 causes a feed-forward cycle and further amplifies and sustains the process. By placing a brake on the system, Klotho protects the heart. Conversely, Klotho deficiency accelerates stress-induced cardiac remodelling. Without stress signals to upregulate TRPC6, neither Klotho deficiency nor overexpression in mice affects cardiac function at baseline. Multiple studies have reported that soluble Klotho inhibits intracellular signalling by insulin and IGF1 [27] , [33] , [34] , [35] . Kurosu et al. [27] first reported that soluble Klotho inhibits insulin and IGF-mediated activation of PI3K pathway by inhibiting activation of receptors and repressing activated receptors. This antiinsulin/IGF effect contributes to aging suppression by Klotho in mice. Wolf et al. further found that soluble Klotho suppresses the growth of human breast and pancreatic cancer cells [33] , [34] . They also found that soluble Klotho coimmunoprecipitated with IGF1 receptors, and suggested that soluble Klotho inhibits the intracellular signalling by IGF1 at least partly by direct interactions with receptors [33] . It was also reported that Klotho prolongs lifespan and stress resistance in C. elegans by blocking insulin and IGF-like signalling in worms [35] . Our results support these previous reports and extend the antiinsulin/IGF role of Klotho to cardioprotection. Cardioprotection by Klotho may contribute to the antiaging effect of Klotho in mice. Activation of PI3K and downstream Akt signalling cascade in the heart is important for physiological cardiac growth, but it can also lead to pathological cardiac hypertrophy [13] , [45] . Inhibition of TRPC6 by soluble Klotho may be a mechanism for preventing PI3K to cause pathological cardiac hypertrophy in the normal heart. Interestingly, shedding of soluble Klotho from membranous Klotho is mediated by metalloproteinases ADAM 10 and 17, and insulin stimulates the shedding through the PI3K pathway [46] . Whether the regulation of shedding of soluble Klotho by insulin/IGF1 has any roles in the control of cardiac functions awaits future investigation. Other TRPC channels including TRPC1, 3, 4 and 5 are also present in the heart. Increased expression of these channels is also associated with cardiac hypertrophy induced by pathological stimuli and downregulation confers the protection [17] , [18] , [19] , [20] . Cardiac TRPC channels are likely heteromultimers of different TRPC members [15] , [22] , [23] , which may partly explain why inhibition of different TRPC channels can confer cardioprotection. The exact molecular composition and stoichiometry of TRPC channels that form heteromultimers with TRPC6 in the heart, however, remains unknown. In this study, deletion of Trpc6 totally abolishes exaggerated ISO-induced cardiac hypertrophy and remodelling in Klotho-deficient mice, indicating that inhibition of TRPC6 alone is sufficient for cardioprotection. Our study yet does not exclude the possibility that soluble Klotho also exerts inhibition on other TRPC channels that form multimers with TRPC6. Of note, Trpc6 deletion only partially blunts ISO-induced hypertrophy, and other factors besides TRPC6 (such as other TRPC channels) are also involved in the hypertrophic response to ISO treatment. Pharmacological TRPC antagonism is in development as a potential treatment of cardiac hypertrophy [21] , [22] , [47] . As an endogenous hormone that may extend human lifespan, soluble Klotho or its analogues or activators [48] may prove to be important therapeutic agents. The involvement of TRPC6 in multiple models of cardiac hypertrophy and heart failure [16] , [17] , [20] and the ability of Klotho to protect against cardiac hypertrophy induced by heart-specific overexpression of TRPC6 suggest that Klotho-based therapeutic strategies may be applicable to diverse cardiac diseases. TRPC6 is also expressed in the kidney, and systemic and pulmonary vasculature, and increased TRPC6 function in these tissues leads to pathologies [15] , [37] , [49] , [50] . Klotho-based therapeutics may also be valuable in treating TRPC6-related pathologies in other organs. One major unanswered question in the pathogenesis of cardiac hypertrophy and remodelling is how the heart distinguishes between overwhelming intracellular calcium transients during each normal cardiac cycle and the abnormal calcium signalling induced by stress signals [44] . Mice with Klotho deficiency or overexpression have no apparent cardiac abnormalities at baseline. The selective targeting to the stress-induced abnormal calcium signalling by Klotho may provide clues to answer this question in the future. General experimental procedures of mice Klotho -hypomorphic, KL-Tg, Trpc6 -knockout, and TRPC6-Tg (line L16) mice have been described [1] , [16] , [27] , [29] . Each mouse line was backcrossed to 129/SvJ mice for >6 generations to achieve congenic background. For dietary phosphate restriction, mice were fed a purified diet containing with 0.2% (wt/wt) inorganic phosphate (TD-09073, Harlan Teklad, Madison, WI) from weaning at ~3 weeks of age. Normal phosphate diets contain 0.35% inorganic phosphate. All mice subjected to experiments were males at ~3 months of age, unless otherwise specified. Blood pressure was measured in WT, Klotho -hypomorphic and KL-Tg mice using a tail-cuff sphygmomanometer as previously described [51] . For induction of cardiac hypertrophy, ISO (2 mg kg −1 per day diluted in PBS) was injected subcutaneously to mice once per day for 10 consecutive days [52] . Control mice received PBS injection. At day 11, mice were euthanized and hearts were isolated. After measurement of weight, a portion of the hearts was snap-frozen in liquid N 2 and saved for RNA isolation, and the remainder fixed and stored for histology. All animal protocols were approved by the University of Texas Southwestern Institutional Animal Care and Use Committee. Real-time quantitative RT–PCR analysis of mRNA RNA was extracted from heart samples with trizol (Invitrogen), reverse-transcribed into cDNA (Taqman reverse transcription reagents, Applied Biosystems-Roche), and mRNA abundance was analysed by real-time PCR with SYBR-green (iTaq or iQ SYBR-green Supermix, BioRad). Primers: GAPDH , 5′-tgcaccaccaactgcttagc-3′, 5′-ggcatggactgtggtcatgag-3′; ANP , 5′-gccatattggagcaaatcct-3′, 5′-gcaggttcttgaaatccatca-3′; BNP , 5′-ccaaggcctcacaaaagaac-3′, 5′-agacccaggcagagtcagaa-3′; β-MHC , 5′-ttggatgagcgactcaaaaa-3′, 5′-gctccttgagcttcttctgc-3′; Trpc6 , 5′-cgctgccaccgtatgg-3′, 5′-ccgccggtgagtcagt-3′. Histological analysis Dissected hearts were rinsed in PBS and incubated in Krebs–Henseleit solution lacking Ca 2+ for 30 min, and were then fixed in 4% paraformaldehyde overnight at room temperature. Samples were dehydrated and stored in 50% ethanol, mounted in paraffin and sectioned. Sections were then stained with haematoxylin and eosin or with Masson’s Trichrome stain. Serum collection and measurement Blood was drawn from mice using retro-orbital bleeding method. Samples were immediately centrifuged, and supernatant collected and stored. Serum phosphate and FGF23 levels were measured using a phosphate assay kit (Stanbio labs, San Antonio, TX) and FGF23 ELISA kit (Kainos lab, Japan), respectively. Cardiac MRI Cardiac MRI of mice was performed in the Mouse MRI Core Facility of UT Southwestern Medical Center as previously described [53] . To determine the LV volume, multiple parallel slices of 1-mm thickness perpendicular to the long heart axis were imaged. The area of LV of each slice at both end-diastolic and end-systolic phases was measured using ImageJ software. LV volume was calculated as the sum of area of all slices at either phase. Stroke volume is the difference between end-diastolic and end-systolic volumes. Ejection fraction is the percentage of stroke volume over end-diastolic volume. Isolation of cardiac ventricular myocyte Isolation of mouse ventricular myocytes was performed per established procedure [54] . Briefly, mice received heparin (100 U per mouse) and anaesthesia. Hearts were quickly removed and perfused retrograde via the aorta with a solution containing (in mM) 113 NaCl, 4.7 KCl, 1.2 MgSO 4 , 0.6 KH 2 PO 4 , 0.6 Na 2 HPO 4 , 10 NaHCO 3 , 30 taurine, 5.5 glucose, 10 2,3-butanedione monoxime, 10 HEPES (at pH 7.4) and followed by a solution containing in addition 1 mg ml −1 type 2 collagenase (Worthinton) and 0.1 mg ml −1 protease XIV (Sigma). The perfusion solution was maintained at 37 °C and equilibrated with 100% O 2 . Thereafter, the ventricle was removed, chopped into small pieces, and further digested in the enzyme solution. After stopping enzyme digestion by adding 2.5% bovine serum albumin and 0.1 mM CaCl 2 , the tissue-cell suspension was filtered through a sterilized-gauze sponge, centrifuged using a tabletop centrifuge at 50 g for 1 min. The resulting cell pellet was resuspended in the stopping buffer and [Ca 2+ ] titrated to 0.5 mM by addition of 100 mM CaCl 2 stock solution in four steps over 20 min. Isolated myocytes were stored at room temperature until use. Whole-cell recording For recording of isolated myocytes, cells were transferred into a perfusion chamber mounted on an inverted microscope and continually perfused at the rate of 1 ml min −1 with bath solution. Whole-cell currents were recorded under voltage-clamp using an Axopatch 200B patch-clamp amplifier (Axon instruments Inc., Foster City, CA, USA) [55] . Voltage protocol consists of holding at −40 mV and repetitive descending ramp pulses from +120 to −120 mV for 500 ms applied every 10 sec. The pipette solution contained (in mM) 9.4 NaCl, 120 CsCl, 1 MgCl 2 , 3.5 CaCl 2 , 10 BAPTA, 10 HEPES, 0.2 NaGTP (pH 7.2) (calculated ionized [Ca 2+ ]~80 nM) and the bath solution contained 140 NaCl, 5 CsCl, 1 MgCl 2 , 1.2 CaCl 2 , 10 glucose, 10 HEPES (pH 7.4). Bath solution also contained 1 μM of nifedipine and 3 mM of NiCl 2 to block current flow through L-type Ca 2+ channel and Na + /Ca 2+ exchanger, respectively. The pipette resistance was ~2–3 MΩ when filled with the pipette solution. Whole-cell access resistance was <10 MΩ. ET-1 (20 nM) was administrated using focal application method. The distance between the tip of the applicator and myocyte was <50 μm. Currents were low-pass filtered at 2 kHz and sampled every 0.1 ms. Data acquisition was performed using pClamp9.2 program (Axon Instrument, Inc.) and analysis using Prism (V3.0) software (GraphPad Software, San Diego, CA, USA). For whole-cell recording of recombinant TRPC6 channels in HEK cells, the pipette and bath solution contained (in mM) 120 Cs-aspartate (Cs-Asp), 10 CsCl, 1 MgCl 2 , 2 MgATP, 5 EGTA, 1.5 CaCl 2 (free [Ca 2+ ]=70 nM) and 10 CsHEPES (pH 7.2) and 140 NaCl, 5 KCl, 0.5 EGTA and 10 NaHEPES (pH 7.4), respectively. Surface biotinylation assay HEK cells expressing haemagglutinin (HA)-tagged TRPC6 (in 35-mm culture dish) were incubated with or without soluble Klotho, washed with 1 ml of ice-cold PBS three times, and incubated with 1 ml of PBS containing 1.5 mg ml −1 EZ-link-NHS-SS-biotin (Thermo Scientific) for 2 h at 4 °C. After quenching with glycine-containing PBS for 20 min, cells were lysed in a buffer (150 mm NaCl, 50 mm Tris–HCl, 5 mm EDTA, 1% Triton X-100, 0.5% deoxycholate and 0.1% SDS) containing protease inhibitor mixture for 30 min. For detection of biotinylated proteins, lysates were precipitated by streptavidin-agarose beads (Thermo Scientific) for 2 h at 4 °C. Beads were subsequently washed three times with TBS containing 1% Triton X-100. Biotin-labelled proteins were eluted in sample buffer, separated by SDS–PAGE, and transferred to nitrocellulose membranes for western blotting using mouse monoclonal anti-HA antibody (Sigma-Aldrich; 1:250 dilution) or anti-α-tubulin antibody (Sigma-Aldrich; 1:500 dilution). Statistical analysis Statistical comparison was made between control and experimental groups conducted during the same time period. Each experiment was repeated at least once at separate times and with similar results. Data are presented as means±s.e.m. Statistical comparison between two groups of data were made using two-tailed unpaired Student’s t -test. Multiple comparisons were determined using one-way analysis of variance followed by Tukey's multiple comparison tests. Statistical comparison of Kaplan–Meier cumulative survival curves was made using ‘log-rank’ analysis ( http://bioinf.wehi.edu.au/software/russell/logrank/ ). How to cite this article: Xie J. et al. Cardioprotection by Klotho through downregulation of TRPC6 channels in the mouse heart. Nat. Commun. 3:1238 doi: 10.1038/ncomms2240 (2012).